Closed network growth of fullerenes Tremendous advances in nanoscience have been made since the discovery of the fullerenes; however, the formation of these carbon-caged nanomaterials still remains a mystery. Here we reveal that fullerenes self-assemble through a closed network growth mechanism by incorporation of atomic carbon and C 2 . The growth processes have been elucidated through experiments that probe direct growth of fullerenes upon exposure to carbon vapour, analysed by state-of-the-art Fourier transform ion cyclotron resonance mass spectrometry. Our results shed new light on the fundamental processes that govern self-assembly of carbon networks, and the processes that we reveal in this study of fullerene growth are likely be involved in the formation of other carbon nanostructures from carbon vapour, such as nanotubes and graphene. Further, the results should be of importance for illuminating astrophysical processes near carbon stars or supernovae that result in C 60 formation throughout the Universe. Fullerenes are efficiently synthesized from graphite by laser ablation or arc-discharge vapourization techniques [1] , [2] , [3] . Despite much investigation since the discovery of Buckminsterfullerene [4] , [5] , [6] , [7] , [8] , [9] , [10] , [11] , [12] , [13] , how these closed cage molecules self-assemble from carbon vapour remains unknown. Proposed fullerene growth models typically invoke small carbon clusters to account for fullerene formation, however, in very different and often conflicting ways [4] , [5] , [6] , [7] , [8] , [11] , [12] . Previous experimental investigations have been unable to differentiate between any of the various bottom-up hypothetical models or identify an alternative mechanism to satisfactorily explain their formation. Recently, a top-down graphene-to-fullerene conversion is even shown to be possible under particular conditions [13] . To exploit the unique mechanical and electrical properties of nanostructured carbon materials such as fullerenes, nanotubes and graphene for use in envisioned paradigm-shifting applications [14] , [15] , [16] , [17] , [18] , [19] , precise control over their formation must be achieved. Such control will only be forthcoming with the revelation of the primary chemical processes that govern their formation. Disclosure of the fullerene growth mechanism is a step toward this ultimate goal. Here we report that fullerenes form bottom-up by ingestion of atomic carbon and small carbon clusters (C 2 ) through a closed network growth (CNG) mechanism. Growth by C and C 2 incorporation is demonstrated for C 60 , C 70 , C 76 , C 78 , C 84 and the endohedral metallofullerenes, La 2 @C 80 and Gd@C 82 . Atomic carbon strongly interacts with the fullerenes during growth and catalyses bond rearrangements. The results open up new experimental approaches for the synthesis or manipulation of fullerenes and nanotubes, and provide fundamental insight into the growth of carbon nanostructures that form under related physicochemical conditions. For example, single-walled carbon nanotubes should also form by CNG [20] , [21] , [22] , [23] , and carbon-catalysed bond rearrangements within graphitic networks open up possible routes toward nanoengineering of carbon materials with precisely tailored structures [24] , [25] . The results also provide insight into fullerene formation in extraterrestrial environments [26] , [27] , [28] . Growth of C 60 in carbon vapour C 60 is one of a large number of fullerenes, which range from around C 30 to hundreds of atoms or more, that spontaneously form in confined carbon vapour produced by the laser ablation of graphite. The short timescale of the growth process and the high-energy conditions of synthesis create severe constraints for experimental investigations of fullerene formation. To overcome these inherent difficulties, we investigate the growth of discrete fullerenes. In the present work, the growth of C 60 and other higher fullerenes is examined by direct exposure to carbon vapour produced from graphite or 13 C-enriched amorphous carbon. Briefly, a fullerene-containing carbon target is subjected to a single laser shot in a pulsed supersonic cluster source ( Fig. 1 ). Upon laser irradiation, the graphite or amorphous carbon target is vapourized into atomic carbon and small clusters, whereas the fullerene is primarily desorbed into this carbon vapour under the flow of helium. The fullerenes then react with carbon vapour, and the species produced then exit the confinement of a clustering zone and undergo a supersonic expansion. The positive ions individually generated from ten such vapourization events are accumulated and then transferred to a high-resolution Fourier-transform ion cyclotron resonance (FT-ICR) mass spectrometer for analysis [29] , and up to three time-domain acquisitions are averaged (see Methods section). The resulting ions are further probed by collision-induced dissociation. The positive ions are expected to be representative of the distribution of neutral fullerenes [1] . 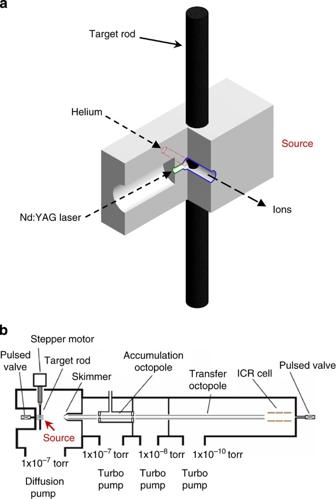Figure 1: Cluster source block and instrument schematic. Cut-away view of cluster source block (a) and instrument schematic (b). A channel 2 mm (red outline) in diameter and ~8.5 mm in length runs from a pulsed valve (70 psi backing pressure) into the region containing the target rod to introduce a flow of helium. A second channel 2 mm (green) in diameter runs orthogonally into the target area to admit the laser beam. A single laser pulse strikes a fullerene-graphite target rod, which desorbs the fullerenes and converts graphite to atomic carbon and C2. Another channel 4 mm (blue) in diameter and ~8.5 mm in length is located downstream from the target, aligned with the helium introduction channel to allow confinement and interaction of the desorbed fullerenes with carbon vapour produced from graphite. After the gas exits this channel, it enters high vacuum and undergoes a free jet expansion. The clusters are then skimmed into octopoles, where ions are accumulated and then transported to the ICR cell for detection. The target rod is simultaneously rotated and translated by a stepper motor. Note: the instrument schematic is not to scale. Figure 1: Cluster source block and instrument schematic. Cut-away view of cluster source block ( a ) and instrument schematic ( b ). A channel 2 mm (red outline) in diameter and ~8.5 mm in length runs from a pulsed valve (70 psi backing pressure) into the region containing the target rod to introduce a flow of helium. A second channel 2 mm (green) in diameter runs orthogonally into the target area to admit the laser beam. A single laser pulse strikes a fullerene-graphite target rod, which desorbs the fullerenes and converts graphite to atomic carbon and C 2 . Another channel 4 mm (blue) in diameter and ~8.5 mm in length is located downstream from the target, aligned with the helium introduction channel to allow confinement and interaction of the desorbed fullerenes with carbon vapour produced from graphite. After the gas exits this channel, it enters high vacuum and undergoes a free jet expansion. The clusters are then skimmed into octopoles, where ions are accumulated and then transported to the ICR cell for detection. The target rod is simultaneously rotated and translated by a stepper motor. Note: the instrument schematic is not to scale. Full size image Laser ablation of pure C 60 in the absence of carbon vapour, Fig. 2a , produces mostly C 60 . C 58 and C 56 are observed at very low relative abundance (and also C 54 , C 52 and C 50 at low abundance) because of fragmentation of the parent C 60 , along with very low abundance clusters larger than C 60 (C 62 to approximately C 72 ). In contrast, remarkable formation of clusters corresponding to C 60+2n results after exposure of C 60 to carbon vapour as shown in Fig. 2b . C 70 is formed at enhanced relative abundance, indicating that the stable isomer obeying the isolated pentagon rule is formed [30] . Fullerenes smaller than C 60 do not form ( Fig. 2b and Supplementary Fig. S1 ), other than from very minor fragmentation of the parent C 60 , suggesting that the growth process is bottom-up. Fragmentation of the larger clusters shows successive loss of C 2 units, a characteristic exclusive to fullerenes, further indicating that these molecular ions are not adducts but are stable fullerene molecules ( Supplementary Fig. S2 ). Coalescence of C 60 to produce species at multiples of C 60 is not observed [31] . In addition, it appears that the cages remain closed during growth, because fullerenes that incorporate the carrier gas, such as He@C 60 or larger He@C 2n , are not observed. He@C 60 is known to form if fullerene cages open at a high pressure of helium at elevated temperature [14] , [32] . 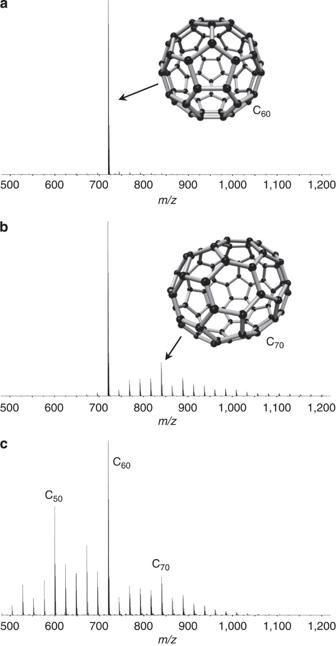Figure 2: FT-ICR mass spectra of laser-ablated C60with and without exposure to carbon vapour. (a) Positive ions produced by laser irradiation of a pure C60target by a single laser pulse at 30–40 mJ cm−2(4.5–6.0 mJ per pulse, Nd:YAG, 532 nm, 3–5 ns, ~1.5 mm beam diameter) in the presence of helium. (b) Larger fullerenes formed by ablation of a C60-graphite target under the same conditions asa. Note: the helium pressure is lower than what is required for fullerene generation from pure graphite. All larger fullerenes formed inbare generated exclusively from gas-phase reactions of desorbed C60with carbon vapour produced from graphite. (c) For comparison, the fullerene distribution produced by ablation of a pure graphite target at a higher helium pressure than inb. Figure 2: FT-ICR mass spectra of laser-ablated C 60 with and without exposure to carbon vapour. ( a ) Positive ions produced by laser irradiation of a pure C 60 target by a single laser pulse at 30–40 mJ cm −2 (4.5–6.0 mJ per pulse, Nd:YAG, 532 nm, 3–5 ns, ~1.5 mm beam diameter) in the presence of helium. ( b ) Larger fullerenes formed by ablation of a C 60 -graphite target under the same conditions as a . Note: the helium pressure is lower than what is required for fullerene generation from pure graphite. All larger fullerenes formed in b are generated exclusively from gas-phase reactions of desorbed C 60 with carbon vapour produced from graphite. ( c ) For comparison, the fullerene distribution produced by ablation of a pure graphite target at a higher helium pressure than in b . Full size image Fig. 2c shows the typical distribution of fullerenes produced by ablation of a pure graphite target, at higher helium pressure than in Fig. 2b . Note that fullerenes smaller than C 60 are formed in high abundance from pure graphite, whereas they are entirely absent when 'growing' C 60 to larger fullerenes upon exposure to carbon vapour. Conversely, the distribution of larger fullerenes (>C 60 ) formed in Fig. 1b and c is essentially duplicated. That similarity supports an identical growth mechanism in both circumstances. To elucidate the growth process, C 60 is exposed to carbon vapour highly enriched in 13 C, shown in Fig. 3 . The desorbed natural isotopic abundance (98.9% 12 C and 1.1% 13 C) C 60 fullerene exhibits monoisotopic 12 C 60 as the most abundant species ( Supplementary Fig. S3 ). After exposure to 13 C-enriched carbon vapour, the C 60 isotopic distribution ( Fig. 3a , left inset) strongly diverges from the natural abundance profile, revealing that 12 C atoms originally present exchange with 13 C atoms [33] , a process that occurs repeatedly. Our calculations show that ingestion of a 13 C atom into the fullerene cage results in 12 C atom ejection, and that atomic carbon simultaneously catalyses bond rearrangements during its interaction with the fullerene, shown in Fig. 4a , confirming previous theoretical predictions that such rearrangements have much more attainable barriers than the pyracylene or Stone-Wales rearrangement [34] . Fig. 4a further shows that the barrier is lower to convert C 2v -C 60 to I h -C 60 (31.0 kcal mol −1 ) rather than convert I h -C 60 to C 2v -C 60 (58.5 kcal mol −1 ) by carbon-catalysed rearrangement. Direct interaction of atomic carbon with fullerenes during growth can thus permit facile bond rearrangements that allow the efficient formation of various fullerene isomers, including the high-symmetry isomers of C 60 and C 70 . Fig. 3b shows that larger fullerene products exhibit isotopic profiles that reveal atom exchange (also see Supplementary Fig. S4 ). 12 C atoms ejected during this process may be subsequently ingested or exchanged with another fullerene, accounting for the deviation from pure 13 C addition (other 12 C sources include approximately 1% 12 C in the amorphous carbon target and possibly 12 C 2 clusters that result from fragmentation). 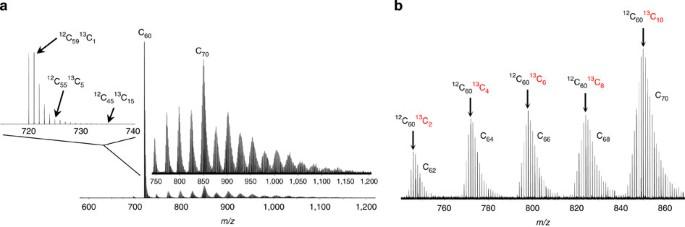Figure 3: Results of exposure of C60to13C-enriched carbon vapour. (a) Positive ions generated from vapourization of a target comprised of amorphous13C (99% atom13C) target mixed with C60under the same conditions as in the C60-graphite experiment (seeFig. 2b), with mass-scale expansion of C60illustrating the occurrence of atom exchange events. (b) C62-C70mass region expanded to show growth of C60to larger fullerenes by successive13C incorporation events. Figure 3: Results of exposure of C 60 to 13 C-enriched carbon vapour. ( a ) Positive ions generated from vapourization of a target comprised of amorphous 13 C (99% atom 13 C) target mixed with C 60 under the same conditions as in the C 60 -graphite experiment (see Fig. 2b ), with mass-scale expansion of C 60 illustrating the occurrence of atom exchange events. ( b ) C 62 -C 70 mass region expanded to show growth of C 60 to larger fullerenes by successive 13 C incorporation events. 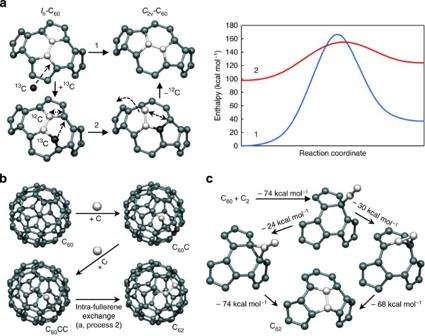Figure 4: Quantum chemical modelling of growth processes. (a) Depictions of C60isomer transformations comparing the conventional Stone-Wales rearrangement (1), and carbon-catalysed bond rearrangement leading to atom exchange (2). The Stone-Wales rearrangement barrier is prohibitive at 164.6 kcal mol−1, whereas the carbon-catalysed bond rearrangement barrier is found to be 58.5 kcal mol−1. (b) C62formation by ingestion of atomic carbon intoIh-C60, followed by structural rearrangement via the mechanism inFig. 4a(process 2). (c) C62formation by ingestion of C2intoIh-C60. Addition of C2to form a 'stick' structure proceeds without a barrier and then further incorporates through the interaction of a [6,6] or [5,6] bond (ΔH=−24 or −30 kcal mol−1). The final step (ΔH=−74 or −68 kcal mol−1) results in C2incorporation across a hexagon with no associated bond rotation to form a heptagon-containing species. Full size image Figure 4: Quantum chemical modelling of growth processes. ( a ) Depictions of C 60 isomer transformations comparing the conventional Stone-Wales rearrangement ( 1 ), and carbon-catalysed bond rearrangement leading to atom exchange (2). The Stone-Wales rearrangement barrier is prohibitive at 164.6 kcal mol −1 , whereas the carbon-catalysed bond rearrangement barrier is found to be 58.5 kcal mol −1 . ( b ) C 62 formation by ingestion of atomic carbon into I h -C 60 , followed by structural rearrangement via the mechanism in Fig. 4a (process 2). ( c ) C 62 formation by ingestion of C 2 into I h -C 60 . Addition of C 2 to form a 'stick' structure proceeds without a barrier and then further incorporates through the interaction of a [6,6] or [5,6] bond ( ΔH =−24 or −30 kcal mol −1 ). The final step ( ΔH =−74 or −68 kcal mol −1 ) results in C 2 incorporation across a hexagon with no associated bond rotation to form a heptagon-containing species. Full size image Fig. 3 conclusively establishes that C 60+2n are formed bottom-up by carbon insertion into C 60 . For example, C 62 predominantly consists of 12 C 60 13 C 2 , which can result only by incorporation of 13 C into the original 12 C 60 desorbed into the 13 C-enriched carbon vapour, formed either through separate atomic 13 C addition steps or by direct 13 C 2 incorporation. Fig. 4b shows C 62 formation by ingestion of atomic carbon into I h -C 60 . Two carbon atoms can separately insert into C 60 to form a C 60 CC species, essentially C 60 with two carbon adatoms. The locations of the two carbon adatoms change as they interchange (without ejection) throughout the C 60 cage by the mechanism shown in Fig. 4a , process 2. Their movement through the fullerene terminates as the adatoms meet to form a bond resulting in a structural conversion to the ground-state fullerene C 62 , the same structure produced by direct C 2 addition. The C 60 CC species can also form by the interaction of two C 60 C species through an inter-fullerene exchange mechanism ( Supplementary Fig. S5 ). We find that direct C 2 ingestion into I h -C 60 proceeds via a series of metastable intermediates, forming a heptagon-containing fullerene as shown in Fig. 4c (see also Supplementary Fig. S6 ). Interestingly, a heptagon-containing C 68 fullerene, although exohedrally stabilized by chlorine, has recently been found to form in carbon vapour [35] . C 64 and all larger clusters possess isotopic distributions that conform to growth by sequential carbon addition steps originating with the C 60 precursor. Effect of laser fluence and carrier gas on C 60 growth Growth to larger fullerenes occurs by uptake of C and C 2 into the C 60 fullerene. Therefore, growth should rely upon parameters that affect interaction between the carbon cages, and C and C 2 , such as carbon-vapour density and length of time of exposure. Carbon density can be controlled by adjusting the laser power; for example, a lower fluence generates less carbon vapour from graphite. The time interval that fullerenes may react with carbon vapour can be roughly controlled by adjusting the helium gas pressure. Inert gas not only confines carbon vapour, but also acts as a carrier gas. A higher flow rate of helium will more quickly push the fullerenes and carbon vapour through the 'clustering zone' (see Fig. 1 ) into vacuum, where they will undergo a supersonic expansion. After that supersonic expansion takes place, all fullerene growth will cease, because a cooled, molecular beam is produced in which very few collisions occur. Thus, vapourization at higher helium pressure can drastically reduce the time interval in which fullerenes may interact with C and C 2 . Fig. 5a shows C 60 exposure to carbon vapour at low laser fluence (7 mJ cm −2 ) and at high helium pressure. The C 60 fullerene, and subsequent larger growth-product fullerenes, incorporates much less carbon. Notably, C 70 does not exhibit any dominance. The distribution directly correlates to what would be expected for CNG by incorporating C and C 2 , rather than larger clusters (C 3 , C 4 , C 5 and so on), under minimal growth conditions. 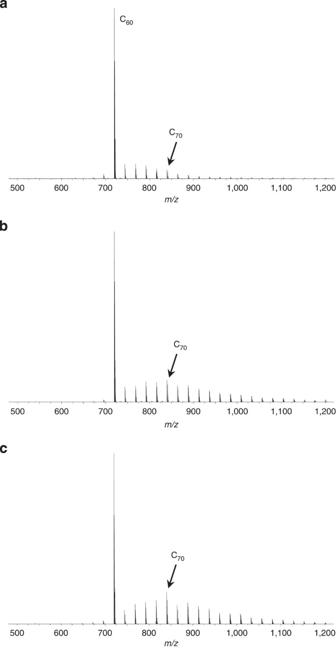Figure 5: Effect of laser fluence and carrier gas on growth. (a) Growth from C60in low carbon-vapour density (laser fluence of 7 mJ cm−2) and high-carrier gas flow rate, which results in conditions that yield minimal interaction with C and C2. Cage growth is minimized and C70does not exhibit an enhanced abundance. (b) Growth from C60at higher carbon-vapour density (laser fluence of 30–40 mJ cm−2), but helium flow rate unchanged froma. More carbon incorporation into C60and a greater abundance of higher fullerenes is observed; however, C70is still not magic-numbered. (c) Carbon density is the same asb, but helium flow rate is slightly decreased, allowing more growth. Larger fullerenes become more abundant, because C60and the newly formed fullerenes interact longer with C and C2, leading to increased carbon incorporation. C70is more abundantly produced. Figure 5: Effect of laser fluence and carrier gas on growth. ( a ) Growth from C 60 in low carbon-vapour density (laser fluence of 7 mJ cm −2 ) and high-carrier gas flow rate, which results in conditions that yield minimal interaction with C and C 2 . Cage growth is minimized and C 70 does not exhibit an enhanced abundance. ( b ) Growth from C 60 at higher carbon-vapour density (laser fluence of 30–40 mJ cm −2 ), but helium flow rate unchanged from a . More carbon incorporation into C 60 and a greater abundance of higher fullerenes is observed; however, C 70 is still not magic-numbered. ( c ) Carbon density is the same as b , but helium flow rate is slightly decreased, allowing more growth. Larger fullerenes become more abundant, because C 60 and the newly formed fullerenes interact longer with C and C 2 , leading to increased carbon incorporation. C 70 is more abundantly produced. Full size image Repeating this experiment at the same helium gas pressure but increasing the laser power (30–40 mJ cm −2 ) produces the growth distribution in Fig. 5b . The fullerenes interact with carbon vapour for the same time interval as in Fig. 5a ; however, the carbon-vapour density is much higher and more collisions between fullerenes, and C and C 2 take place, resulting in enhanced growth. Finally, Fig. 5c shows the distribution of larger fullerenes produced after exposure of C 60 to carbon vapour at the same laser fluence in Fig. 5b , but the helium pressure is slightly reduced. Hence, the amount of time the fullerenes interact with carbon vapour is increased. Accordingly, more ingestion of C and C 2 takes place, which results in greater growth to larger fullerenes. The newly formed fullerenes have more time to interact with atomic carbon, which allows the most stable isomers, such as isolated pentagon rule D 5h -C 70 , to form by the carbon-catalysed bond rearrangements shown in Fig. 4a . The most stable fullerene isomers are more resistant to carbon incorporation and will exhibit an increase in abundance. We note that carbon-catalysed bond rearrangements can transform the original I h -C 60 to a more reactive isomer, such as C 2v -C 60 (ref. 36 ). The C 2v -C 60 isomer contains fused pentagons, resulting in more highly pyramidalised carbon atoms that are more susceptible to reaction with carbon. Consequently, the observed fullerenes are not necessarily the direct fullerene isomer that leads to most growth. In addition, regarding growth from pure graphite, I h -C 60 is not likely to be formed directly from its C 58 fullerene precursor, but may be easily converted to it by the carbon-catalysed bond rearrangements. C 60 growth using hydrogen as an in situ probe It has been previously shown that vapourization of graphite in the presence of hydrogen inhibits fullerene production [37] . In fact, fullerene formation is found to completely cease upon vapourizing graphite at a high pressure of hydrogen gas. The interpretation is that, because hydrogen is very reactive, any 'dangling bonds' of carbon structures react rapidly with it, interrupting a critical growth stage. Polycyclic aromatic hydrocarbons are mostly formed rather than fullerenes. Therefore, hydrogen may be used as an in situ probe to further decipher if the hollow cages grow by addition to dangling carbon bonds, and thus open structures, or via CNG. C 60 is exposed to carbon vapour with hydrogen gas as shown in Fig. 6 . Growth of C 60 in a high pressure of hydrogen gas, Fig. 6a , essentially reproduces the growth distribution in which helium is used ( Fig. 5b ). It is clear that hydrogen does not terminate or disrupt the growth process. Growth by cage opening via reactive dangling bonds is inconsistent with this observation. By contrast, the result is consistent with closed cage growth. 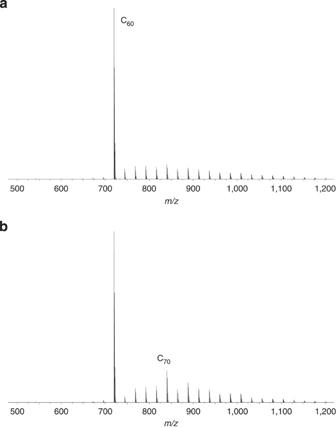Figure 6: C60growth in hydrogen. (a) C60exposed to carbon vapour with pure hydrogen gas at high pressure. Growth to larger fullerenes is revealed showing that the reactive fullerene intermediates remain closed cages. (b) At slightly lower hydrogen flow rate, C70becomes special, and it is clearly shown that the same growth processes occur as when helium is used, further demonstrating that the growth process occurs via carbon addition to closed networks. Figure 6: C 60 growth in hydrogen. ( a ) C 60 exposed to carbon vapour with pure hydrogen gas at high pressure. Growth to larger fullerenes is revealed showing that the reactive fullerene intermediates remain closed cages. ( b ) At slightly lower hydrogen flow rate, C 70 becomes special, and it is clearly shown that the same growth processes occur as when helium is used, further demonstrating that the growth process occurs via carbon addition to closed networks. Full size image Repeating the experiment at lower pressure, Fig. 6b , shows that C 70 becomes dominant. The dominance of C 70 suggests carbon-catalysed bond rearrangement is still possible in the presence of hydrogen. Quantum chemical calculations for bond rotation between C 2v -C 60 -CH and I h -C 60 -CH found a barrier of 52.4 kcal mol −1 (see Supplementary Fig. S7 ), demonstrating that a hydrogenated carbon adatom is nearly as efficient at catalysing bond rearrangements as its non-hydrogenated equivalent. Fullerene growth from pure graphite is drastically affected by the presence of hydrogen, because the dangling carbon bonds of non-caged structures that initially form the smallest fullerenes are terminated with hydrogen, significantly disrupting formation. Our results clearly demonstrate that a preformed cage is able to grow to larger fullerenes in the presence of pure hydrogen, entirely consistent with the closed-cage reactive intermediates of a CNG mechanism. CNG of endohedral metallofullerenes Endohedral fullerenes continue to be a widely researched, exciting class of nanomaterial. However, even less is known about the formation of these fullerenes that trap atoms within the cage [38] . Importantly, the demonstration of growth for an endohedral metallofullerene can provide crucial experimental confirmation that the fullerene cages must remain closed during incorporation of C and C 2 , because the internally located atoms will be lost if the cage opens [14] . The encapsulated metal acts as another in situ probe to characterize the growth mechanism. La 2 @C 80 , comprised of an I h -C 80 cage encapsulating two freely rotating lanthanum atoms [14] , is exposed to carbon vapour generated from graphite. Fig. 7a shows that growth to much larger La 2 @C 80+2n metallofullerenes (>La 2 @C 120 ) is clearly exhibited after exposure of La 2 @C 80 to carbon vapour. The larger growth product ions fragment by C 2 loss with retention of both La atoms, confirming that the larger La 2 @C 2n species are endohedral metallofullerenes ( Supplementary Fig. S8 ). Recently, La 2 @C 100 has been structurally characterized, revealing a nanotubular carbon network [39] . The large metallofullerene, Sm 2 @C 104 , has also been shown to possess a tubular structure [40] . Therefore, the La 2 @C 80+2n growth-product fullerenes may exist as essentially small nanotubes, and prolonged exposure to carbon vapour should further extend their size. 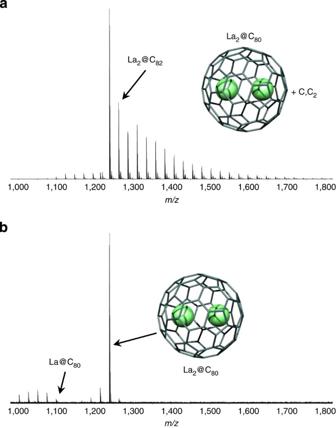Figure 7: CNG of endohedral metallofullerenes. (a) Larger La2@C2nendohedral fullerenes are formed after exposure of La2@C80to carbon vapour by laser ablation (50 mJ cm−2) of a La2@C80-coated graphite target. (b) Laser irradiation (50 mJ cm−2) of La2@C80without exposure to carbon vapour. An encapsulated La atom can be ejected to form La@C80and C2loss-fragment ions. When exposed to carbon vapour, this small amount of La@C80formed will grow by the CNG mechanism (rather than fragment) to produce the very weak La@C2nsignals ina. Figure 7: CNG of endohedral metallofullerenes. (a ) Larger La 2 @C 2n endohedral fullerenes are formed after exposure of La 2 @C 80 to carbon vapour by laser ablation (50 mJ cm −2 ) of a La 2 @C 80 -coated graphite target. ( b ) Laser irradiation (50 mJ cm −2 ) of La 2 @C 80 without exposure to carbon vapour. An encapsulated La atom can be ejected to form La@C 80 and C 2 loss-fragment ions. When exposed to carbon vapour, this small amount of La@C 80 formed will grow by the CNG mechanism (rather than fragment) to produce the very weak La@C 2n signals in a . Full size image Almost all growth clusters observed in Fig. 7a are endohedral metallofullerenes that contain two La atoms. Very weak abundances of La@C 2n and extremely weak abundances of C 2n are also observed ( Supplementary Fig. S9 ). Those weakly observed signals of fullerenes are present because of the creation and subsequent growth of La@C 80 and C 80 , resulting from fragmentation of La 2 @C 80 . Fig. 7b shows La 2 @C 80 laser ablated under the same conditions as in Fig. 7a , but not exposed to carbon vapour. The behaviour of that fullerene after interaction with the highly energetic laser beam can be determined. It is clear that most of the La 2 @C 80 remains completely intact; however, a very small portion of La 2 @C 80 fragments by C 2 loss. As a result of that fragmentation process, loss of a single La atom to form La@C 80 (and C 2 loss fragment ions, La@C 80 -C 2n ), and an even smaller percentage lose both La atoms to form empty cage C 80 (and C 2 loss fragment ions, C 80 -C 2n ), is observed. That same fragmentation process of the parent La 2 @C 80 will occur when exposed to carbon vapour, because the same laser fluence is used in both Fig. 7a and b (also see Supplementary Fig. S10 ). However, when exposed to carbon vapour, La@C 80 and C 80 will not fragment by C 2 loss, but will instead grow via CNG to larger fullerenes to form the weakly observed La@C 2n and extremely weak C 2n signals. Nevertheless, it is unequivocally demonstrated that almost all growth occurs with retention of both the La atoms, which confirms closed cage growth. The metallofullerene, Gd@C 82 , is also demonstrated to grow via carbon insertion into a closed cage ( Supplementary Figs S11, S12 and S13 ), further confirming the CNG mechanism. Growth of higher fullerenes The extent of incorporation of carbon further increases upon exposure of C 60 to carbon vapour in the absence of helium, and at an even higher laser fluence as shown in Fig. 8a . Moreover, enhanced relative abundances for 'magic number' species are observed under these conditions and become even more evident as larger fullerenes are probed. Notably, much more C 70 is formed from C 60 under these growth conditions. The enhanced growth results from maximum fullerene residence time in the confines of the clustering zone, and therefore more interaction with carbon vapour, because of the absence of carrier gas. The increased laser fluence creates a higher-density carbon vapour that promotes more carbon insertion that results in enhanced growth to larger fullerenes. Even in the absence of helium, a supersonic expansion still takes place, which permits the gas to be transported into the ion optics for accumulation and transfer to the ICR cell for detection. 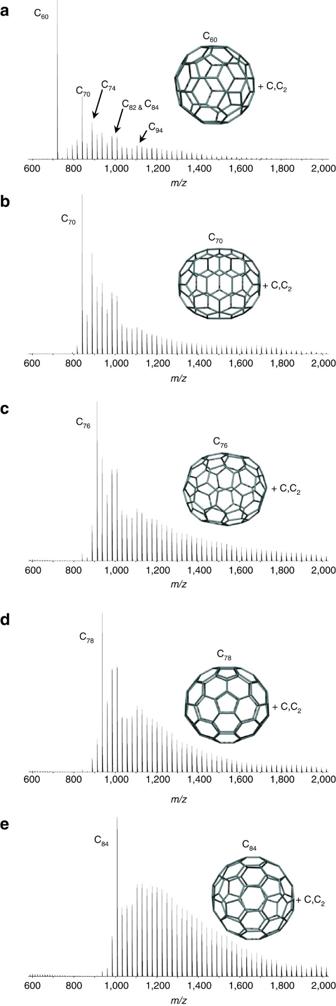Figure 8: Growth of higher fullerenes. Growth of Ih-C60(a), D5h-C70(b), C76(c), C78(d), and C84(e). In absence of carrier gas and at higher laser fluence (60–90 mJ cm−2), the fullerenes incorporate more C and C2, and the 'magic number' clusters exhibit enhanced abundances. Smaller fullerenes are not observed, except from minor fragmentation of the parent fullerene during laser irradiation, and it is unequivocally revealed that C60is not formed from the growth processes of higher fullerenes.Ih-C60is also demonstrated to be the most resistant toward carbon incorporation. Note: what appears to be weak signals in the m/z 600–800 range forc–eare spectral artifacts (second harmonics, at half the mass-to-charge ratio), because of the larger growth cluster cations that are formed in greater abundance because the isomers of C76, C78and C84are much more reactive to C and C2ingestion thanIh-C60orD5h-C70. Figure 8: Growth of higher fullerenes. Growth of Ih-C 60 ( a ), D5h-C 70 ( b ), C 76 ( c ), C 78 ( d ), and C 84 ( e ). In absence of carrier gas and at higher laser fluence (60–90 mJ cm −2 ), the fullerenes incorporate more C and C 2 , and the 'magic number' clusters exhibit enhanced abundances. Smaller fullerenes are not observed, except from minor fragmentation of the parent fullerene during laser irradiation, and it is unequivocally revealed that C 60 is not formed from the growth processes of higher fullerenes. I h -C 60 is also demonstrated to be the most resistant toward carbon incorporation. Note: what appears to be weak signals in the m/z 600–800 range for c – e are spectral artifacts (second harmonics, at half the mass-to-charge ratio), because of the larger growth cluster cations that are formed in greater abundance because the isomers of C 76 , C 78 and C 84 are much more reactive to C and C 2 ingestion than I h -C 60 or D 5h -C 70 . Full size image The fullerenes C 70 , C 76 , C 78 and C 84 were independently probed under the same growth conditions ( Fig. 8b–e ). The distribution of clusters formed by exposure of C 70 to carbon vapour reproduces the >C 70 distribution in Fig. 8a exhibited by growth of C 60 . We have confirmed that the larger growth species are not present in the purified fullerene starting materials ( Supplementary Fig. S14 ). Regardless of the choice of fullerene starting materials, the same magic number fullerene (C 74 , C 82 , C 84 , C 92 ) trends are observed. Thus, fullerene growth proceeds along a single mechanistic path. The observations further confirm bottom-up growth by ingestion of C and C 2 , because the same magic-number fullerenes would not likely form if incorporation of larger clusters (C 3 , C 4 , C 5 and so on) were a significant process. Importantly, these results show that I h -C 60 , and also to some extent D 5h -C 70 , are significantly less reactive toward carbon ingestion than other fullerenes, explaining the dominant production of C 60 from graphite. Note that the distributions of fullerenes formed under these conditions bear a striking resemblance to those produced in sooting flames [41] . That observation suggests that the same CNG mechanism applies to fullerene formation in sooting flames and other synthesis methods that involve generation of C or C 2 , although the initial formation mechanism of the smallest fullerene may differ. The CNG mechanism appears to potentially have a broad, unifying reach. Fig. 8 unequivocally demonstrates that CNG of higher fullerenes (C 70 , C 76 , C 78 , C 84 ) do not result in the production of C 60 . Consequently, C 60 formation is a result of CNG from smaller fullerenes. Further, we do not observe any small fullerenes (<C 50 ) in our growth investigations. Those findings are consistent with the conjecture that the smallest fullerenes are the first to form and serve as precursors to C 60 (and all larger fullerenes) during synthesis from pure graphite [7] . Inert gas, such as helium, appears to be crucial overall for the formation of fullerenes from pure graphite, but its presence is clearly not required for growth once a fullerene is formed. Therefore, it appears that inert gas is essential only for the efficient formation of the smallest fullerene, which once formed, grows rapidly by carbon ingestion to larger fullerenes via the CNG mechanism. The presence of inert gas may allow for the highest possible carbon-vapour density, which in turn permits formation of the smallest fullerene. It may also allow the clustering process to more readily proceed by permitting three body collisions to form C 3 , after which the growth to all larger clusters (and eventually the smallest fullerene) can proceed by two body collisions [7] . A possible initial formation mechanism regarding how the smallest fullerene may form has been previously demonstrated by the coalescence of cyclic carbon species, which can exist in carbon vapour under fullerene-generating conditions [9] . The long-standing problem regarding how I h -C 60 forms in such high abundance from carbon vapour is resolved. I h -C 60 is simply a 'bottleneck' in the closed-cage growth process. We have experimentally demonstrated that fact by comparing the growth of I h -C 60 to C 70 , C 76 , C 78 and C 84 . The results demonstrate that endohedral fullerenes also form by CNG and provide the first clear insight into their formation as well. The encapsulated atoms or moieties must be placed within the fullerene cage upon initial formation of the smallest endohedral fullerene, and they may catalyse or nucleate endohedral fullerene formation. It may now be possible to design synthetic strategies that allow for more efficient production of endohedral fullerenes and incorporation of new chemical units. Moreover, exposure of preformed endohedral metallofullerenes to carbon vapour may provide a more efficient avenue to access and discover new large fullerenes. We observe the formation of nanostructures much larger than C 250 after exposure of C 60 and other fullerenes to carbon vapour. Therefore, the growth process appears to have no upper limit. It is likely that these larger structures are nanotubular rather than spheroidal. Fullerenes, nanotubes and graphene can all be synthesized by various carbon vapour techniques. Questions now arise as to whether C and C 2 can interact in a similar way with the carbon networks of other nanostructures. For example, carbon nanotubes contain 'fullerene endcaps', and it seems highly plausible that C and C 2 addition by the CNG mechanism would occur at such sites. Further, the results strongly suggest that extension in length of a preformed carbon nanotube can be realized by exposure to carbon vapour to create an extremely long tube. C 60 was originally discovered in experiments designed to probe carbon chemistry in the outflows of carbon stars. The recent discovery of C 60 and C 70 in space illustrates that the processes we disclose in this study could be of direct importance to their possible formation in the environments of carbon stars or supernovae [26] , [27] , [28] . The CNG mechanism provides a clear route for the formation of fullerenes in the presence of hydrogen. Therefore, the results are likely to be valuable for further deciphering fullerene formation in extraterrestrial environments. 9.4 T FT-ICR mass spectrometry All experiments are analysed with a custom-built FT-ICR mass spectrometer based on a 9.4 T, 155 mm bore diameter actively shielded superconducting magnet, and were performed with positive ions. The cluster source is housed in a source chamber (1×10 −7 torr) evacuated by a 3,000 l s −1 diffusion pump. The vapourization of the target rod is achieved by a single laser shot (pulse) fired from an Nd:YAG (532 nm, 3–5 ns, 0.5–13.5 mJ per pulse, ~1.5 mm beam diameter) laser via a quartz window, in conjunction with the opening of the pulsed valve (800 μs pulse width). The timing of the laser shot is adjusted to coincide with a desired helium pressure within the source. A shot fired later in time after the maximum of the pulsed valve pressure profile will irradiate the target under lower helium pressure. The helium pressure in the growth experiments is below the narrow range to produce fullerenes directly from graphite. The ions produced in the cluster source are transported to the ICR cell via three stages of differential pumping, each supplied with a turbomolecular pump to achieve ultrahigh vacuum (10 −10 torr) in the ICR cell. After exiting the clustering region, the ions are skimmed into an octopole ion guide (175 V p−p , 1.8 MHz, 570 mm length) and immediately transferred to a second octopole for ion accumulation. Ions are confined radially in the accumulation octopole (240 V p−p , 2.8 MHz, 160 mm) by a time-varying electric field generated by a radiofrequency applied with 180° phase difference to adjacent rods and axially by the application of positive voltages to the end caps at the conductance limits at either side of the accumulation octopole. Helium gas is introduced through a pulsed valve to the accumulation octopole (~10 −4 torr) to facilitate further cooling. After the accumulation of ions produced by ten individual laser and helium-pulse events, the ions are transferred by a third octopole (155 V p−p , 2.2 MHz, 1450 mm) to an open cylindrical ion trap (70 mm diameter, 212 mm, aspect ratio ~2) [42] . The ions are accelerated to a detectable cyclotron radius by a broadband frequency sweep excitation (260 V p−p , 150 Hz μs −1 , 3.6–0.071 MHz) and subsequently detected as the differential current induced between two opposed electrodes of the ICR cell. Each of the acquisitions is Hanning-apodised and zero-filled once before fast Fourier transform and magnitude calculation [43] . Up to three time-domain acquisitions are averaged. The experimental event sequence is controlled by a modular ICR data acquisition system [44] . Ions are further probed by collision-induced dissociation. Sustained off-resonance irradiation collision-induced dissociation Ions of interest are isolated by applying a SWIFT (stored waveform inverse Fourier transform) event [45] . The selected ions are then subjected to a 10-ms pulse of helium directly injected into the ICR cell via a pulsed valve located outside the magnet bore, followed by 250 μs single frequency excitation at 1 KHz off-resonance [29] . After a 15- to 20-s delay to allow the system to re-establish base pressure, a broadband frequency sweep is performed before detection. The mass spectrum is obtained from a single time-domain acquisition. Fullerene samples I h -C 60 (99.9%), D 5h -C 70 (>99%), C 76 (mixture of isomers, 99.5%), C 78 (mixture of isomers, >99%), C 84 (mixture of isomers, >99%), La 2 @ I h -C 80 (>99%), Gd@ C 2v -C 82 (~98%). C 60 and C 70 were purchased commercially. All other fullerene samples are synthesized by arc discharge and purified by multistage high-performance liquid chromatography [46] . Preparation of fullerene-graphite target Fullerene (500 μg) is dissolved in a minimal amount of carbon disulfide or toluene and uniformly applied to a preheated graphite rod (99.999%). After further heating at 250°C for several minutes, the rod is placed in the high-vacuum source chamber at base pressure (10 −7 torr) for several hours before use to ensure removal of all solvent. A new graphite rod is used for each experiment. Preparation of fullerene- 13 C amorphous carbon target C 60 (500 μg) is mixed with 5 mg of 13 C-enriched amorphous carbon (99% atom 13 C). A layer of the powdered mixture is mechanically applied to the surface of a 6.3-mm diameter ground quartz rod. Preparation of fullerene films A solution of 500 μg fullerene in minimal amount of solvent is applied to a 6.3-mm diameter ground quartz rod, with heating (250°C) during application for several minutes. The coated quartz rod is then placed into the high-vacuum source. The removable source block and quartz rods are meticulously cleaned and then immersed in H 2 O 2 /H 2 SO 4 mixture after each experiment to ensure that all carbonaceous material is completely removed. Calculations Density Functional Theory within the Local Density Approximation was performed by use of the AIMPRO package [47] , [48] . The charge density was fitted to plane waves with an energy cut-off of 200 Ry. Charge density oscillations in partly filled degenerate orbitals during the self-consistency cycle were damped by use of a Fermi occupation function with kT =0.04 eV. Relativistic pseudo-potentials [49] were used for all atoms. Atom-centered Gaussian basis functions were used to construct the many-electron wave function, with angular momenta up to l =2, with 22 independent functions per carbon atom. A Bloch sum of these functions is performed over the lattice vectors to satisfy the periodic boundary conditions of the supercell. A large cubic supercell ( a =21.17 Å) was used to ensure no interaction with neighbouring fullerenes. Calculations were performed with a single k-point (½,½,½). Lowest energy spin states were determined, and for all calculations spin zero was employed except for isolated C 2 , which was 0.47 eV more stable in the triplet state, and the C 60 C 2 'stick' structure, which was only stable in the triplet state. Reaction barriers were determined with the climbing nudged elastic band method [50] with either 12 or 24 intermediate structures. How to cite this article : Dunk, P. W. et al . Closed network growth of fullerenes. Nat. Commun . 3:855 doi: 10.1038/ncomms1853 (2012).